TET2lesions enhance the aggressiveness ofCEBPA-mutant acute myeloid leukemia by rebalancingGATA2expression The myeloid transcription factor CEBPA is recurrently biallelically mutated (i.e., double mutated; CEBPA DM ) in acute myeloid leukemia (AML) with a combination of hypermorphic N-terminal mutations ( CEBPA NT ), promoting expression of the leukemia-associated p30 isoform, and amorphic C-terminal mutations. The most frequently co-mutated genes in CEBPA DM AML are GATA2 and TET2 , however the molecular mechanisms underlying this co-mutational spectrum are incomplete. By combining transcriptomic and epigenomic analyses of CEBPA - TET2 co-mutated patients with models thereof, we identify GATA2 as a conserved target of the CEBPA - TET2 mutational axis, providing a rationale for the mutational spectra in CEBPA DM AML. Elevated CEBPA levels, driven by CEBPA NT , mediate recruitment of TET2 to the Gata2 distal hematopoietic enhancer thereby increasing Gata2 expression. Concurrent loss of TET2 in CEBPA DM AML induces a competitive advantage by increasing Gata2 promoter methylation, thereby rebalancing GATA2 levels. Of clinical relevance, demethylating treatment of Cebpa-Tet2 co-mutated AML restores Gata2 levels and prolongs disease latency. Acute myeloid leukemia (AML) is characterized by genetic alterations affecting the proliferation and/or differentiation of hematopoietic stem or progenitor cells (HSPCs). Thereby, the expansion of immature myeloid precursors, at the expense of normal hematopoiesis, ultimately leads to bone marrow (BM) failure if left untreated. Recent sequencing efforts have identified numerous recurrent mutations in AML and revealed patterns of mutational co-segregation, suggesting that synergism between certain lesions drives leukemogenesis [1] . While we now recognize these patterns, the mechanistic basis for context-specific positive or negative selection of certain lesions remains to be elucidated in most cases. CCAAT enhancer binding protein alpha (CEBPA) is a hematopoietic lineage-specific transcription factor that binds and primes genes for myeloid development and is required for differentiation and maturation of granulocytes [2] . The gene encoding CEBPA is biallelically mutated (i.e., double mutated; CEBPA DM ) in 3–15% of de novo AML patients [3] , [4] , [5] , [6] , [7] , [8] , [9] . CEBPA DM patients harbor either biallelic N-terminal mutations or a combination of a monoallelic N-terminal mutation together with a C-terminal mutation in the other allele. Whereas N-terminal CEBPA ( CEBPA NT ) lesions promote the expression of the truncated p30 isoform, C-terminal mutations result in CEBPA variants that are unable to dimerize or bind DNA, thus rendering them inactive. Hence, CEBPA p30 homodimers are the sole entity with functional transcription factor activity in CEBPA DM AML. This is in contrast to normal hematopoietic cells where the full-length p42 isoform is predominantly expressed [2] . CEBPA p30 lacks two of three transactivation elements present in p42, but retains one transcriptional activating element and the basic-region leucine-zipper, which enables dimerization and DNA-binding [10] . CEBPA p30 has functions distinct from CEBPA p42 and can bind an isoform-specific set of enhancers and regulate the expression of downstream effector genes, such as Nt5e and Msi2 [11] , [12] . Importantly, in the context of CEBPA DM AML, the CEBPA NT is hypermorphic, leading to higher levels of the transcription factor, and thus, increased binding to enhancers and subsequent deregulation of gene expression [11] . In line with these data, mice with CEBPA p30 expression driven from the endogenous Cebpa locus develop AML with full penetrance within a year [13] . Most patients with CEBPA DM AML also feature additional mutations in GATA2 , TET2 , WT1 , NRAS , FLT3 , or CSF3R [9] . Several of these mutations are found together with CEBPA DM more frequently than expected by the individual frequency of each mutation, while other combinations are statistically underrepresented. Recent studies have shed light on the molecular mechanisms underlying mutational cooperativity for some of the co-mutated genes, i.e. GATA2 [14] and CSF3R [15] , while mechanistic insight is still lacking for other subgroups of CEBPA DM AML. Of particular importance are mutations in the gene encoding the methylcytosine dioxygenase TET2 which, by converting 5-methylcytosine to 5-hydroxymethylcytosine, promotes DNA demethylation. TET2 mutations ( TET2 MUT ) are frequent in CEBPA DM AML cases and are associated with inferior prognosis [16] , [17] . Moreover, loss of Tet2 has been implicated in accelerating and/or aggravating hematological malignancies in combination with several other recurrent gain-of-function and loss-of-function mutations [18] , [19] , [20] , reflecting the importance of appropriately regulated DNA demethylation in normal hematopoiesis. Importantly, while Tet2 loss alone only mildly affects hematopoiesis with myeloid skewing and increased competitiveness of HSCs [18] , as well as the increased propensity of leukemic blasts to switch to a more stem-like phenotype [21] , it does not induce overt leukemia per se [22] , [23] , [24] . Despite being extensively studied, mechanistic insights of how TET2 loss-of-function cooperates with other aberrations have been hampered by the fact that malignant cells have been compared to their normal, wild-type counterparts in many studies. In the present work, we sought to overcome this limitation by comparing CEBPA- mutant AML in the presence and absence of additional mutations in TET2 . By combining transcriptomic and epigenomic analyses of relevant in vitro and in vivo models as well as data from AML patients, we identified an intricate mechanism where TET2 loss-of-function rebalances Gata2 expression levels in Cebpa DM AML, and hence drives an aggressive disease. TET2 mutations impair outcome for patients with CEBPA -mutant AML To validate previous reports on the spectrum of co-occurring mutations in CEBPA DM AML patients, we compiled data from 557 CEBPA DM cases and evaluated the co-occurrence of other known leukemia driver mutations [3] , [4] , [5] , [6] , [7] , [17] . TET2 was the second most frequently co-mutated gene, with 1 in 5 CEBPA DM cases harboring TET2 mutations (Fig. 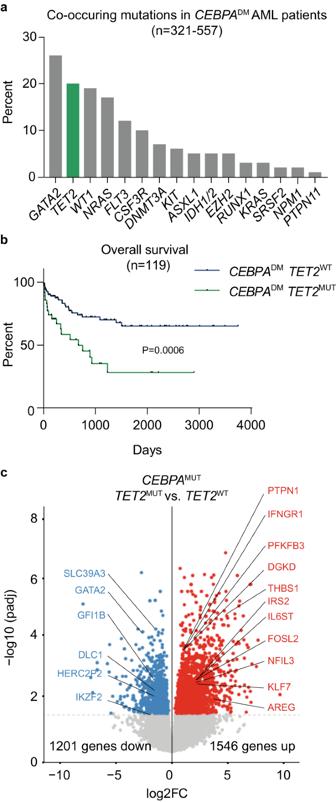Fig. 1:TET2mutations impair outcome for patients withCEBPA-mutant AML. aFrequency of co-occurring mutations inCEBPADMAML cases, data aggregated from published cohorts3,4,5,6,7,8,17(321–557 cases; detailed in Supplemental Table1).bOverall survival ofCEBPADMpatients with wild-type (TET2WT; 84 patients) or mutatedTET2(TET2MUT; 35 patients). The data were analyzed by Mantel-Cox Log-rank test.cVolcano plot depicting differentially expressed genes dependent onTET2mutational status in the cohort ofCEBPA-mutant patients in the Beat AML dataset (TET2WT11 andTET2MUT5 patients). Differential analysis was performed with DESeq2 (P< 0.05). Source data are provided as a Source Data file. 1a ; Supplemental Table 1 ). Importantly, the survival of TET2 -mutant ( TET2 MUT ) CEBPA DM patients was significantly lower than TET2 wild-type ( TET2 WT ) CEBPA DM patients (Fig. 1b ), consistent with previous reports [16] , while the presence of TET2 mutations did not cause a higher overall number of mutations in CEBPA DM patients (Supplemental Fig. 1a ). Fig. 1: TET2 mutations impair outcome for patients with CEBPA -mutant AML. a Frequency of co-occurring mutations in CEBPA DM AML cases, data aggregated from published cohorts [3] , [4] , [5] , [6] , [7] , [8] , [17] (321–557 cases; detailed in Supplemental Table 1 ). b Overall survival of CEBPA DM patients with wild-type ( TET2 WT ; 84 patients) or mutated TET2 ( TET2 MUT ; 35 patients). The data were analyzed by Mantel-Cox Log-rank test. c Volcano plot depicting differentially expressed genes dependent on TET2 mutational status in the cohort of CEBPA -mutant patients in the Beat AML dataset ( TET2 WT 11 and TET2 MUT 5 patients). Differential analysis was performed with DESeq2 ( P < 0.05). Source data are provided as a Source Data file. Full size image To investigate the functional consequences of TET2 and CEBPA co-mutations, we analyzed RNA sequencing (RNA-seq) data from the Beat AML dataset [1] . We identified 1546 up- and 1201 downregulated genes in patients harboring a combination of CEBPA and TET2 mutations when compared to CEBPA -mutant patients with wild-type TET2 (Fig. 1c ). Similarly, a slight overrepresentation of up-regulated genes was observed when comparing CEBPA WT TET2 MUT patients to CEBPA WT TET2 WT patients (601 up- and 527 downregulated). In line with the lower overall survival of TET2 MUT CEBPA DM patients, pathways related to inflammation, hypoxia, and aggressive cancer were upregulated in CEBPA-TET2 co-mutated patients (Supplemental Fig. 1b ). The overrepresentation of up-regulated genes associated with TET2 deficiency in CEBPA MUT (and CEBPA WT ) patients is somewhat surprising, as increased DNA methylation upon TET2 loss would be expected to cause global transcriptional repression. However, other co-occurring mutations and residual DNA demethylase activity from the TET2 WT allele may cause a more complex pattern of gene expression. These findings indicate that mutations in TET2 enhance the aggressiveness of CEBPA -mutant AML by deregulation of critical cellular pathways. TET2 deficiency accelerates Cebpa -mutant AML To study the effect of TET2 mutations in CEBPA DM AML in pathophysiologically relevant in vitro and in vivo models, we utilized cell and murine models in which expression of the p30 isoform is retained ( Cebpa p30/p30 or Cebpa Δ/p30 ), while the normal p42 isoform of CEBPA is completely lost [13] . Since TET2 is predominantly inactivated by loss-of-function mutations [25] , we modeled TET2 mutations either by the introduction of mutations with the CRISPR-Cas9 technology or by conditional knockout of the Tet2 alleles. First, we introduced Tet2 mutations into a murine myeloid progenitor cell model ( Cebpa p30/p30 ) (Fig. 2a ). Tet2 -targeted cells displayed a selective advantage, as they outcompeted Cebpa p30/p30 cells (Fig. 2b ). Detailed analysis of the Tet2 mutation that was associated with the proliferative advantage showed that the Tet2 locus had acquired a + 1 insertion in exon 3, which resulted in a downstream premature termination codon (Supplemental Fig. 2a, b ). In line with this, clones isolated from the targeted cell pool exhibited strongly reduced TET2 protein expression (Supplemental Fig. 2c ). Gene expression analysis revealed that Tet2 loss in Cebpa p30/p30 cells caused downregulated expression of 916 genes, while only 540 genes were upregulated (Fig. 2c ). Gene set enrichment analysis (GSEA) showed higher expression of MYC and E2F targets in Cebpa p30/p30 Tet2 -mutated cells, consistent with their proliferative advantage (Supplemental Fig. 2d ). Fig. 2: TET2 deficiency accelerates Cebpa -mutant AML. a Schematic representation of generation of Tet2 -knockout clones with CRISPR/Cas9. The illustration was created with BioRender.com. b Proliferative outgrowth of Cebpa p30/p30 cells with Tet2 indels. c Volcano plot depicting differentially expressed genes dependent on the Tet2 mutational status in Cebpa p30/p30 cells ( Tet2 WT 7 and Tet2 MUT 5 clones). Differential analysis was performed with DESeq2 ( P < 0.05). d Experimental setup for evaluating the effect of Tet2 -deficiency ( Tet2 Δ/Δ ) in Cebpa DM AML initiation in vivo. The illustration was created with BioRender.com. e Myeloid (Mac1 + ) contribution of donor-derived blood and bone marrow (BM) cells evaluated after BM transplantation and Cre-LoxP recombination. (Blood samples: Week 12; 6 mice per group. Week 24; Cebpa Δ/p30 Tet2 +/+ and Cebpa +/Δ Tet2 Δ/Δ 6 mice per group and Cebpa +/Δ Tet2 Δ/Δ 3 mice. Week 36; 3 mice per group. BM samples: 3 mice per group.) Data are presented as mean±SEM and analyzed by one-way-ANOVA followed by Dunnett’s multiple comparisons correction. f Survival of lethally irradiated recipient mice after BM transplantation and Cre-LoxP recombination ( Cebpa Δ/p30 Tet2 +/+ 12 mice, Cebpa Δ/p30 Tet2 Δ/Δ 14 mice, and Cebpa +/- Tet2 Δ/Δ 14 mice). The data were analyzed by Mantel-Cox Log-rank test. g Volcano plot depicting differentially expressed genes dependent on Tet2 deficiency status in Cebpa Δ/p30 leukemic blasts (samples from 3 mice per group). Differential analysis was performed with DESeq2 ( P < 0.05). h Frequency of proliferating (Ki67 + ) cells in BM of moribund recipient mice (specimens from 3 mice per group). Data are presented as mean±SEM and analyzed by a two-tailed unpaired t -test. Source data are provided as a Source Data file. Full size image In summary, these data show that CRISPR/Cas9-induced TET2 loss provides a competitive advantage to myeloid progenitors expressing the oncogenic CEBPA variant p30. Next, we wanted to assess the impact of hematopoietic expression of CEBPA p30 ( Cebpa Δ/p30 ) with TET2-deficiency ( Tet2 −/− ) on AML initiation in vivo. To do so, we transplanted lethally irradiated recipient mice with BM cells derived from mice with relevant allele combinations and, following hematopoietic reconstitution, induced hematopoietic-specific knockout of the Cebpa WT allele and/or the Tet2 alleles (Fig. 2d ). The combination of CEBPA p30 expression with Tet2 loss led to an early expansion of myeloid (Mac1 + ) cells in the BM and blood compared to mice with hematopoietic cells featuring either alteration on its own (Fig. 2e ; Supplemental Fig. 2e ). Conforming to patient data and data obtained from Cebpa p30/30 cells, Cebpa Δ/p30 Tet2 Δ/Δ hematopoietic cells gave rise to AML with shorter latency than Cebpa Δ/p30 Tet2 +/+ cells, with a median survival of 23 and 43 weeks, respectively (Fig. 2f ). Mice transplanted with Cebpa Δ/p30 Tet2 +/+ BM cells developed leukemia with similar latency as mice transplanted with Cebpa p30/p30 fetal liver cells [13] . This is consistent with the matching expression of Cebpa in these two contexts (1.1 ± 0.24 vs. 1.0 ± 0.13 (relative expression) in Cebpa p30/p30 and Cebpa Δ/p30 Tet2 +/+ AML blasts n = 3/group, respectively). TET2 deficiency alone ( Cebpa Δ/+ Tet2 Δ/Δ ) did not give rise to AML and cells which retained expression of the p42 isoform from one allele ( Cebpa +/p30 ) only sporadically underwent leukemic transformation, in line with unaltered Cebpa expression levels in these cells (Fig. 2f ; Supplemental Fig. 2f ; 1.03 ± 0.14 vs. 1.0 ± 0.04 (relative expression) in Cebpa fl/p30 and Cebpa fl/+ cells n = 2–3/group, respectively). The transformed blasts expressed myeloid (Mac1 + ) and granulocytic (Gr1 + ) markers, confirming the myeloid origin of the leukemia (Supplemental Fig. 2g ). The leukemias were transplantable into secondary recipients, and the shorter latency of the TET2-deficient Cebpa DM AML was preserved in this setting (Supplemental Fig. 2h–i ), indicating that TET2 not only has important tumor suppressive functions during malignant transformation but also during progression of AML. We performed RNA-seq on Cebpa Δ/p30 ( Tet2 WT and knockout) AML blasts to assess changes in gene expression upon TET2 deficiency. Again, we found that the majority of differentially expressed genes was decreased in TET2-deficient AML blasts, with 176 down- vs. 58 upregulated genes (Fig. 2g ). GSEA highlighted upregulation of genes involved in IL-6-JAK-STAT-signaling and hypoxia, in line with RNA-seq data from human TET2 MUT CEBPA MUT cases (Supplemental Fig. 1b ; Supplemental Fig. 2j ). Furthermore, pathways related to cell cycle progression (G2M checkpoint and E2F targets) were enriched in TET2-deficient AML, indicating increased growth upon loss of TET2, consistent with the effects observed in the cell model (Supplemental Fig. 2d ; Supplemental Fig. 2j ). In line with this, we found that a higher frequency of Cebpa Δ/p30 Tet2 Δ/Δ blasts expressed the proliferation marker Ki67 (Fig. 2h ). In addition, we also observed increased proliferative capacity of Cebpa Δ/p30 Tet2 Δ/Δ blasts compared to Cebpa Δ/p30 Tet2 +/+ blasts ex vivo. This difference was dependent on Tet2 status, as the TET2 co-factor Vitamin C was able to mitigate proliferation of Cebpa Δ/p30 Tet2 +/+ but not of Cebpa Δ/p30 Tet Δ/Δ cells (Supplemental Fig. 2k ). Collectively, these data show that TET2 deficiency accelerates the establishment and progression of CEBPA p30-driven AML in vivo. Loss of TET2 leads to reduced Gata2 levels in Cebpa -mutant AML To find conserved gene targets of the CEBPA-TET2 axis, we integrated the transcriptomic data from our in vitro and in vivo models with gene expression analyses from AML patients harboring CEBPA and TET2 mutations. Three target genes exhibited downregulated expression in all three data sets; FUT8 , GATA2 , and SIRT5 (Fig. 3a ; Supplemental Fig. 3a–c ). Fig. 3: Loss of TET2 leads to reduced Gata2 levels in Cebpa -mutant AML. a Conserved targets of the CEBPA-TET2 axis visualized in a Venn-diagram of downregulated genes in CEBPA - TET2 co-mutated AML overlaid with corresponding data from Tet2 -deficient in vivo and in vitro models of Cebpa DM AML ( P = 0.0264 vs. number of overlapping genes expected by random distribution assessed by Wilson/Brown binominal test). b Heatmap of differentially accessible regions assessed by assay for transposase-accessible chromatin sequencing (ATAC-seq; FDR < 0.05), and c genomic distribution of downregulated peaks (FDR < 0.05, Log2FC < 0) upon Tet2 mutation (4 clones per group). Differential analysis was performed with DiffBind and region enrichment analysis with GREAT. d Representative genome wide DNA-methylation status in leukemic blasts from the in vivo model assessed by whole genome bisulfite sequencing (WGBS) showing frequency of methyl-cytosine (mC) across the transcription start site (TSS) ±1000 base pairs, gene body scaled to 4000 base pairs, and transcription termination site (TES) ±1000 base pairs. Methylation analysis was performed with Bismark and visualized using deepTools. e Median and interquartile range of percent mC at promoters of down- ( n = 172), not expressed ( n = 6539), not differentially expressed (not DE; n = 14759) and up-regulated ( n = 57) genes (averaged data generated from 2 Cebpa Δ/p30 Tet2 +/+ and 3 Cebpa Δ/p30 Tet2 Δ/Δ mice). Whiskers indicates max–min and data were analyzed by two-tailed unpaired t -test. f Promoter DNA methylation of conserved target genes in leukemic blast (samples from 2 Cebpa Δ/p30 Tet2 +/+ and 3 Cebpa Δ/p30 Tet2 Δ/Δ mice). Data are presented as mean±SEM. The data were log-transformed and analyzed by two-tailed unpaired t -test. g Gata2 variant mRNA expression in Cebpa Δ/p30 Tet2 Δ/Δ and Cebpa Δ/p30 Tet2 +/+ leukemic blasts (samples from 3 mice per group). Data are presented as mean ± SEM. The data were log-transformed and analyzed by a two-tailed unpaired t -test. h Schematic genomic view of the Gata2 locus, including representative examples of assay for transposase-accessible chromatin using sequencing (ATAC-seq) in Cebpa p30/p30 cells. Source data are provided as a Source Data file. Full size image Since the deregulation of these three genes was observed across species and differential experimental setups, we next aimed to investigate if their decreased gene expression was a direct result of TET2 deficiency. We therefore assessed chromatin accessibility and DNA methylation as a proxy for TET2 binding and activity [26] . Through assay for transposase-accessible chromatin sequencing (ATAC-seq), we identified 1809 differentially accessible regions in Cebpa p30/p30 Tet2 MUT vs. Cebpa p30/p30 Tet2 WT cells, and consistent with an activating effect of TET2, the majority of differential regions were less accessible in TET2-deficient cells (Fig. 3b ). Half of the ATAC-seq peaks downregulated upon Tet2 mutation were located in promoters, and these regions were enriched for GATA and NFAT motifs (Fig. 3c ; Supplemental Fig. 3d ). Using whole genome bisulfite sequencing (WGBS), we observed a global increase in DNA methylation in Cebpa Δ/p30 Tet2 Δ/Δ vs. Cebpa Δ/p30 Tet2 +/+ AML blasts, consistent with a loss of demethylase activity in Tet2 knockout blasts (Fig. 3d ). Increased DNA methylation was observed in promoter regions of genes whose expression were downregulated upon TET2 loss ( + 54%; Fig. 3e ), while upregulated and not differently expressed genes did not show any marked changes. Strikingly, this pattern was not apparent when DNA methylation was evaluated across gene bodies (Supplemental Fig. 3e ). Non-expressed genes exhibited equal increase in DNA methylation across promoters and gene bodies (Fig. 3e ; Supplemental Fig. 3e ). Since increased gene body methylation is not associated with gene repression [27] , we evaluated whether a gain in gene body methylation was coupled to a gain in promoter methylation for the down-regulated genes. In the presence of promoter hypermethylation, the bodies of down-regulated genes were more prevalently hypermethylated compared to neutral and up-regulated genes (34.8% [95%CI 18.8–55.11] vs. 18.1% [16.4–19.9], p = 0.0427). While, in the absence of promoter hypermethylation, the bodies of up-regulated genes tended to be hypermethylated compared to neutral and down-regulated genes (13.8% [95%CI 7.2–24.9] vs. 7.1% [6.8–7.4], p = 0.0518). Thus, loss of TET2 in Cebpa DM cells caused decreased chromatin accessibility and increased methylation of DNA in promoters of TET2-responsive genes, consistent with previous reports showing that TET2 binding is enriched in promoters of TET2-regulated genes [28] . To identify direct CEBPA-TET2 gene target(s), we evaluated the previously identified conserved candidates based on changes in DNA methylation of their promoters. Out of the three target genes, only the gene encoding the transcription factor GATA-binding factor 2 (GATA2) showed a gain of DNA methylation in the promoter of the gene variant 2 ( Gata2 V2 ) upon TET2 deficiency ( + 46%; Fig. 3f ). In line with this, specifically the Gata 2 V2 mRNA isoform was downregulated in TET2-deficient Cebpa DM AML blasts (−86%; Fig. 3g ), while changes in mRNA expression and promoter methylation of Gata2 V1 did not reach statistical significance (Fig. 3f, g ). In summary, these analyses identify Gata2 (locus overview in Fig. 3h ) as a conserved target of the CEBPA-TET2 axis across several settings. TET2 deficiency causes increased DNA methylation of the Gata2 promoter, resulting in reduced mRNA expression. Moderate Gata2 reduction increases competitiveness of Cebpa -mutant AML GATA2 is an essential transcription factor for hematopoietic cells and has profound effects on HSC maintenance. Moreover, it is recurrently mutated in AML [29] , [30] and GATA2 lesions are overrepresented in CEBPA DM AML [8] , [16] , [31] , [32] , [33] . Given these critical roles of GATA2, we next examined the consequences of reduced GATA2 levels in CEBPA DM AML. To test if reduced Gata2 expression would provide a competitive advantage in vivo, we set up an RNA-interference (RNAi) based competition assay (Fig. 4a ) utilizing established Cebpa p30/p30 leukemia cells, in which both Cebpa (+56–73%) and Gata2 (+45–56%) levels are increased modestly compared to primary Cebpa Δ/p30 Tet2 +/+ blasts [11] , [34] . First, we identified four short hairpin RNAs (shRNA) which lowered Gata2 expression to a varying degree (Fig. 4b ). Upon transplantation of shRNA-expressing cells, we observed a non-monotonic relationship between Gata2 expression levels and competitiveness, as measured by sh Gata2 -to-shControl ratios. While efficient downregulation of Gata2 expression did not provide any competitive advantage to Cebpa DM cells, moderate silencing imposed a three-fold increase in their ability to compete (Fig. 4c, d ). Repetition of this experiment including only the most and least efficient shRNAs in a separate experiment yielded similar results (Supplemental Fig. 4a, b ). These results were mirrored by increased expression of the proliferation marker Ki67 in cells expressing the least efficient Gata2 -targeting shRNA but not the most efficient one (Supplemental Fig. 4c ). To test if the same effects are observed in an in vitro setting, we targeted Gata2 in Cebpa p30/p30 cells using the CRISPR/Cas9 approach. Gata2 -targeted cells showed a proliferative advantage over Gata2 WT cells, leading to their outgrowth (Fig. 4e, f ). In accordance with previously published data that complete loss of Gata2 expression results in a loss of competitiveness [35] , [36] , [37] , we found that only clones with heterozygous Gata2 inactivation were viable, while clones with homozygous mutations in Gata2 could not be recovered (Supplemental Fig. 4d ). Fig. 4: Moderate Gata2 reduction increases competitiveness of Cebpa- mutant AML. a Experimental setup for evaluating the effect of Gata2 knockdown, via short hairpin RNA (shRNA) mediated silencing, on Cebpa p30/p30 leukemic cells in a competitive in vivo assay. The illustration was created with BioRender.com. b Gata2 mRNA in Cebpa p30/p30 leukemic cells prior to transplantation. c Representative flow cytometry profiles of input and output of shControl (no knockdown), sh Gata2 A (low knockdown), and sh Gata2 D (high knockdown). d Competitive advantage of targeting shRNA (GFP + ) vs. non-targeting shRNA (YFP + ) cells in vivo assessed as by flow cytometry (Control 4, sh Gata2 A 4, sh Gata2 B 4, sh Gata2 C 4, and sh Gata2 D 3 mice). Data are presented as mean±SEM. Data were log-transformed and analyzed by one-way-ANOVA followed by Dunnett’s multiple comparisons correction. e Experimental setup for Gata2 CRISPR/Cas9 mutagenesis in Cebpa p30/p30 cells, and outgrowth of heterozygous mutated clones. Percentages of Gata2 mutated clones are indicated. f Growth curve of Cebpa p30/p30 clones with Gata2 mutation ( Cebpa p30/p30 Gata2 +/MUT , n = 10) or wild type Gata2 ( Cebpa p30/p30 Gata2 +/+ , n = 3). Data are presented as mean±SEM and analyzed by two-tailed unpaired t -test. Red lines mark individual mutated clones. 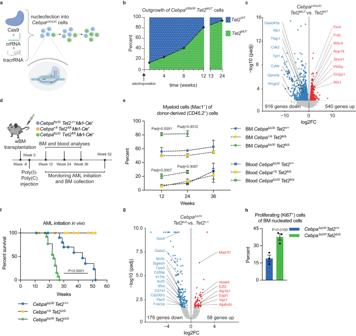Fig. 2: TET2 deficiency acceleratesCebpa-mutant AML. aSchematic representation of generation ofTet2-knockout clones with CRISPR/Cas9. The illustration was created with BioRender.com.bProliferative outgrowth ofCebpap30/p30cells withTet2indels.cVolcano plot depicting differentially expressed genes dependent on theTet2mutational status inCebpap30/p30cells (Tet2WT7 andTet2MUT5 clones). Differential analysis was performed with DESeq2 (P< 0.05).dExperimental setup for evaluating the effect ofTet2-deficiency (Tet2Δ/Δ) inCebpaDMAML initiation in vivo. The illustration was created with BioRender.com.eMyeloid (Mac1+) contribution of donor-derived blood and bone marrow (BM) cells evaluated after BM transplantation and Cre-LoxP recombination. (Blood samples: Week 12; 6 mice per group. Week 24;CebpaΔ/p30Tet2+/+andCebpa+/ΔTet2Δ/Δ6 mice per group andCebpa+/ΔTet2Δ/Δ3 mice. Week 36; 3 mice per group. BM samples: 3 mice per group.) Data are presented as mean±SEM and analyzed by one-way-ANOVA followed by Dunnett’s multiple comparisons correction.fSurvival of lethally irradiated recipient mice after BM transplantation and Cre-LoxP recombination (CebpaΔ/p30Tet2+/+12 mice,CebpaΔ/p30Tet2Δ/Δ14 mice, andCebpa+/-Tet2Δ/Δ14 mice). The data were analyzed by Mantel-Cox Log-rank test.gVolcano plot depicting differentially expressed genes dependent onTet2deficiency status inCebpaΔ/p30leukemic blasts (samples from 3 mice per group). Differential analysis was performed with DESeq2 (P< 0.05).hFrequency of proliferating (Ki67+) cells in BM of moribund recipient mice (specimens from 3 mice per group). Data are presented as mean±SEM and analyzed by a two-tailed unpairedt-test. Source data are provided as a Source Data file. g Presence or absence of GATA2 mutations ( GATA2 MUT ) in CEBPA double mutated ( CEBPA DM ) AML cases with or without TET2 mutations ( TET2 MUT ) in aggregated data from published cohorts [3] , [4] , [5] , [7] , [8] , [17] (detailed in Supplemental Table 2a ). Data were analyzed by Wilson/Brown binominal test. Source data are provided as a Source Data file. Full size image If the pro-leukemogenic effect of TET2 mutations was, at least partly, caused by lowering GATA2 expression, we reasoned that concomitant mutations in both genes would be redundant and thus, the pattern of TET2 and GATA2 mutations would be mutually exclusive. Indeed, TET2 MUT CEBPA DM AML cases showed a lower frequency of GATA2 mutations than expected from the frequency of GATA2 mutations in TET2 WT CEBPA DM AML cases (Fig. 4g ; Supplemental Table 2a ), which was also true for all AML cases (3.5% in TET2 MUT vs. 8.9% in TET2 WT ; Supplemental Fig. 4e ; Supplemental Table 2b ). Importantly, whereas mutations in WT1 followed the same pattern as TET2 , CSF3R mutations appeared in equal frequency between TET2 MUT CEBPA DM and TET2 WT CEBPA DM AML cases, and ASXL1 mutations were increased in TET2 MUT CEBPA DM AML (Supplemental Fig. 4f ; Supplemental Table 2c–e ). While we favor a functional redundancy model, we cannot exclude that co-mutation of TET2 and GATA2 could induce synthetic lethality in AML cells, as Gata2 -loss has been shown to induce terminal myeloid differentiation [37] . Altogether, our data suggest that loss of TET2 in Cebpa DM AML causes a moderate decrease in Gata2 expression, which in turn increases the competitive fitness of the leukemia. Hence, this indicates that TET2 and GATA2 mutations are partially redundant in CEBPA DM AML, providing a mechanistic rationale for the mutational spectrum observed in this AML entity. Increased CEBPA p30 binding to the Gata2 distal hematopoietic enhancer drives expression of Gata2 via TET2 We next asked if GATA2 expression is dependent on CEBPA mutational status. To this end, we exploited published transcriptomics data from human and mouse CEBPA DM AML [11] . GATA2 expression was increased in human CEBPA DM leukemic granulocyte/monocyte progenitors (GMPs) compared to GMPs from healthy donors ( + 77%; Supplemental Fig. 5a ). Correspondingly, Gata2 was upregulated in murine Cebpa p30/p30 leukemic GMPs as compared to normal GMPs ( + 43%; Fig. 5a ). Likewise, analysis of AML patient data from the BEAT AML study [1] , revealed that both CEBPA and GATA2 expression were increased in CEBPA NT AML compared to CEBPA WT AML ( + 91% and +37%, respectively), while GATA2 expression was reverted to CEBPA WT level in CEBPA NT TET2 MUT AML ( Supplemental Fig. 5b, c ). Since CEBPA is known to exert its transcription factor activity by binding to enhancers and thereby promote gene expression [38] , we assessed the binding of CEBPA to the crucial Gata2 distal hematopoietic enhancer ( G2 DHE; −77 kb in mouse) that governs Gata2 expression in hematopoietic stem and progenitor cells including GMPs [11] , [39] . Notably, we found substantially increased levels of CEBPA bound to the G2 DHE in Cebpa p30/p30 leukemic GMPs compared to their normal counterparts ( + 147%; Fig. 5b ), while the binding levels associated with other known proximal and distal cis- regulatory elements of the Gata2 gene were unchanged (Supplemental Fig. 5d, e ). Additionally, TET2 showed significant binding to the G2 DHE in Cebpa p30/p30 cells (Fig. 5c ). However, DNA methylation at the G2 DHE was low and unaltered upon Tet2 loss (Supplemental Fig. 5f ). Importantly, CEBPA binding, as assessed by ChIP-qPCR, was not altered by introduction of Tet2 mutations in Cebpa p30/p30 cells (Supplemental Fig. 5g ). Fig. 5: Increased CEBPA p30 binding to the Gata2 distal hematopoietic enhancer drives expression of Gata2 via TET2. a Gata2 mRNA expression in mouse Cebpa p30/p30 leukemic granulocyte/monocyte progenitors (GMPs) vs normal GMPs (samples from 4 Cebpa +/+ and 2 Cebpa p30/p30 mice) and, b CEBPA binding to the Gata2 distal hematopoietic enhancer ( G2 DHE; −77 kb) region (samples from 2 mice per group), data from Jakobsen et al. [11] . Data are presented as mean ± SEM. Differential analysis was performed with DESeq2 ( P < 0.05). c Schematic genomic view of the Gata2 distal hematopoietic enhancer ( G2 DHE), including normalized chromatin immunoprecipitation sequencing (ChIP-seq) signal of CEBPA (data from Heyes et al. [12] ), TET2 and H3K27Ac (data from Heyes et al. [12] ), as well as assay for transposase-accessible chromatin using sequencing (ATAC-seq) in Cebpa p30/p30 cells without (light blue) and with (green) mutation in Tet2 . d Gata2 mRNA levels in response to targeting of the G2 DHE by CRISPR-Cas9 in Cebpa p30/p30 cells in vitro using indicated sgRNAs and e the averaged change in Gata2 mRNA levels of the 12 deletions (averaged data from 2 separate experiments). Data are presented as median ± range and analyzed by two-tailed Wilcoxon signed-rank test. f Experimental setup for evaluating the effects of Cebpa knockout on Gata2 V2 mRNA expression and DNA methylation of the CpG island at the promoter of Gata2 V2 in MLL-fusion driven AML ( iMLL-AF9 ). The illustration was created with BioRender.com. g Gata2 V2 mRNA expression (leukemic cell lines generated from 2 separate mice were assayed on 2 separate days in 2–3 technical replicates each). Data are presented as mean ± SEM and the individual cell lines are indicated by circles or squares. Data were log-transformed and analyzed by two-tailed unpaired t -test. h DNA methylation of the Gata2 V2 promoter CpG-island (2 separate leukemic cell lines). Data are presented as median±range and the individual cell lines are indicated by circles or squares. i Experimental setup for evaluating the effects of Cebpa knockdown on TET2 binding to the G2 DHE in Cebpa p30/p30 cells with inducible expression of shRNA targeting Cebpa and control ( Renilla ), respectively. The illustration was created with BioRender.com. j TET2 binding to the G2 DHE assessed by ChIP-qPCR (3 replicates per condition). Data are presented as mean±SEM and analyzed by two-tailed unpaired t -test. k Frequency of GATA2 and/or TET2 mutations ( GATA2 MUT and TET2 MUT , respectively) in CEBPA high expressing ( CEBPA HIGH ; 45 cases) vs. CEBPA low expressing (CEBPA LOW ; 61 cases) AML cases, data from Beat AML cohort [1] . The distributions of GATA2 WT TET2 WT vs. GATA2 MUT and/or TET2 MUT cases were analyzed by Wilson/Brown binominal test. Source data are provided as a Source Data file. Full size image These results prompted us to test if CEBPA binding to the G2 DHE modulates Gata2 expression in Cebpa DM AML. We deleted 250–500 bp fragments of the Gata2 enhancer encompassing the CEBPA binding site using the CRISPR/Cas9 approach in Cebpa p30/p30 cells in vitro. Expression of total Gata2 mRNA, as well as both individual transcript variants, was decreased upon targeting the genomic region with strong CEBPA binding compared to non-targeting control (Fig. 5c–e , Supplemental Fig. 5h–k ). In contrast, Gata2 expression was unchanged when G2 DHE deletions were introduced in Cebpa p30/p30 Tet2 MUT cells (Supplemental Fig. 5l, m ). Combined, these data suggest that CEBPA binding to the G2 DHE is important for promoting Gata2 expression in Cebpa DM AML. Further, the G2 DHE has been shown to primarily regulate expression of the hematopoietic specific Gata2 variant 2 ( V2 ) [40] , [41] , conforming with our data that particularly the Gata2 V2 promoter displayed an increase in DNA methylation and that the Gata 2 V2 mRNA was downregulated in TET2-deficient Cebpa DM AML blasts (Fig. 3f–g ). Next, we tested if the reduction of CEBPA in AML cells influenced the expression and promoter DNA methylation of Gata2 V2 . Given the dependence of CEBPA DM AML on CEBPA for survival and maintenance, we utilized MLL-fusion-driven AML, in which CEBPA is dispensable for the maintenance of established leukemia [42] . Cre-mediated loss of Cebpa in leukemic cells expressing the inducible MLL-AF9 fusion-protein ( iMLL-AF9 + Cebpa Δ/Δ ; Fig. 5f ) caused reduced Gata2 V2 mRNA levels compared to control cells ( iMLL-AF9 + Cebpa fl/fl ) ( − 72%; Fig. 5g ). Importantly, the methylation frequency of the CpG island located at the Gata2 V2 promoter was increased in two separate leukemic lines ( + 186%; Fig. 5h ; Supplemental Fig. 5n ), suggesting that Gata2 V2 mRNA expression is regulated via the CEBPA-TET2 axis. Finally, we assessed TET2 binding to the G2 DHE upon Cebpa knockdown in Cebpa p30/p30 cells using ChIP-qPCR (Fig. 5i ). Notably, we observed decreased TET2 binding to the G2 DHE in cells expressing sh Cebpa compared to cells expressing control shRNA, verifying that CEBPA is important for recruitment of TET2 to the G2 DHE (Fig. 5j ). In light of these findings, we asked whether elevated CEBPA level and not the CEBPA mutation(s) per se, drives the selective pressure for GATA2 and/or TET2 loss in AML to achieve moderate GATA2 levels that are optimal for leukemia growth. We therefore stratified AML cases in the Beat AML cohort [1] based on CEBPA expression and assessed their GATA2 and TET2 mutational status. Indeed, the frequency of GATA2 and/or TET2 mutations was three-fold higher in CEBPA HIGH AML compared to the CEBPA LOW samples (Fig. 5k ). In line with previous data showing a hypermorphic effect of CEBPA DM [11] , the CEBPA HIGH group contained the majority of the CEBPA -mutant cases in the cohort (82 and 100% of CEBPA SM and CEBPA DM , respectively), while none of the cases in the CEBPA LOW group were CEBPA -mutated. In conclusion, our data show that elevated CEBPA binding to the G2 DHE, driven by the hypermorphic effect of Cebpa NT , increases TET2-mediated demethylation of the Gata2 promoter, which leads to elevated Gata2 levels in Cebpa DM AML. In this context, Cebpa DM AML cells gain a competitive advantage by loss of TET2, which in turn promotes an increase in DNA methylation at the Gata2 promoter resulting in the rebalancing of Gata2 levels. Demethylating treatment restores Gata2 expression and prolongs survival in TET2-deficient Cebpa -mutant AML Finally, we investigated if treatment with the demethylating agent 5-azacytidine (5-AZA) would be beneficial in TET2-deficient CEBPA DM AML. Ex vivo treatment with 5-AZA restored Gata2 expression in Cebpa Δ/p30 Tet2 Δ/Δ blasts to levels observed in Cebpa Δ/p30 Tet2 +/+ , while 5-AZA treatment did not affect Gata2 levels in Cebpa Δ/p30 Tet2 +/+ cells (Supplemental Fig. 6a ). Moreover, 5-AZA decreased the viability of blasts from both genotypes, although to a higher degree in the TET2-deficient setting (−82% and −40%, respectively, p < 0.01; Supplemental Fig. 6b ). To evaluate if the enhanced effect of 5-AZA treatment in TET2-deficient AML would also hold true in vivo, mice were transplanted with Cebpa Δ/p30 Tet2 Δ/Δ or Cebpa Δ/p30 Tet2 +/+ AML blasts and treated with 5-AZA for three consecutive days after disease establishment (Fig. 6a ). While the blast frequency of TET2-deficient Cebpa Δ/p30 AML decreased upon 5-AZA treatment ( − 62%; Fig. 6b ), the treatment did not significantly decrease the frequency of TET2-proficient cells. Furthermore, 5-AZA treatment restored Gata2 levels in Cebpa Δ/p30 Tet2 Δ/Δ blasts in vivo to the same level as in Cebpa Δ/p30 Tet2 +/+ blasts (Fig. 6c ). Intriguingly, two out of three individual Cebpa Δ/p30 Tet2 Δ/Δ leukemic clones (A + B) responded to 5-AZA treatment with a pronounced increase of Gata2 levels and concomitant reduction of myeloid blasts, while one clone (C) appeared partially refractory to 5-AZA treatment, with limited increase of Gata2 and no reduction of leukemic burden (Fig. 6b, c ). Importantly, a longer intermittent 5-AZA treatment prolonged the survival of mice transplanted with Cebpa Δ/p30 Tet2 Δ/Δ blasts from one of the responding clones (A) (median survival +22%; Fig. 6d, e ), while it did not affect disease latency of mice transplanted with Cebpa Δ/p30 Tet2 +/+ blasts (A). Fig. 6: Demethylating treatment restores Gata2 expression and prolongs survival in TET2-deficient Cebpa -mutant AML. a Experimental setup for evaluating the effect of short-term 5-azacytidine (5-AZA) treatment in vivo. Recipient mice were sub-lethally irradiated and transplanted with leukemic BM from moribund secondary recipient mice. Three individual Cebpa Δ/p30 Tet2 Δ/Δ clones (A–C) and two Cebpa Δ/p30 Tet2 +/+ clones (A–B) were used, respectively. The illustration was created with BioRender.com. b Expansion of myeloid (Mac1 + ) donor-derived cells in bone marrow (BM) assessed by flow cytometry, and c Gata2 mRNA expression in sorted leukemic blasts by qPCR assessed 24 hours after the last of three injections of 5-AZA or vehicle (samples from 3 mice per clone and 6 and 9 mice per group, for Cebpa Δ/p30 Tet2 +/+ and Cebpa Δ/p30 Tet2 Δ/Δ , respectively). Dot plots showing individual mice for separate clones and bar graphs shows mean ± SEM for each group. Data were analyzed by Kruskal–Wallis test followed by Dunn’s correction for multiple comparisons. d Experimental setup for evaluating the effect of 5-AZA treatment on AML progression in vivo. The illustration was created with BioRender.com. e Survival of sub-lethally irradiated tertiary recipient mice after transplantation of leukemic BM from moribund secondary recipient mice (clone A from both genotypes) in response to intermittent 5-AZA treatment (5-AZA treated groups 8 mice and vehicle-treated groups 4 mice). The data were analyzed by Mantel–Cox Log-rank test. Source data are provided as a Source Data file. Full size image In summary, we show that the demethylating agent 5-AZA can restore Gata2 expression levels in TET2-deficient Cebpa DM AML to that of TET2-proficient Cebpa DM AML, and concomitantly reduce leukemic burden and prolong survival of mice transplanted with TET2-deficient Cebpa DM leukemic blasts. Mutational cooperativity is a fundamental driver of cancer development, progression, and aggressiveness. For CEBPA DM AML, co-occurring lesions have been found in genes such as GATA2 , TET2 , WT1 , FLT3 , and CSFR3 . While the mechanistic basis for the cooperation between CEBPA and GATA2/CSFR3 mutations has been investigated using mouse models [14] , [15] , we have very little insight into why other lesions, such as those in TET2 , are overrepresented in CEBPA DM AML. Here, we show that TET2 loss-of-function in CEBPA DM AML leads to an aggressive disease phenotype by rebalancing the increased and suboptimal levels of GATA2 that are induced by hypermorphic CEBPA NT mutations driving CEBPA-p30 isoform expression (see model in Fig. 7a ). Specifically, loss of TET2 binding to the hematopoietic-specific G2 DHE enhancer results in increased DNA methylation in the promoter region of the hematopoietic-specific Gata2 isoform ( Gata2 V2 ). This proleukemic effect of TET2 loss can be reversed by the demethylating agent 5-AZA, suggesting that this could be a potential treatment option in CEBPA DM TET2 MUT patients. Altogether, our work proposes that CEBPA-mutant AMLs acquire additional lesions in genes such as GATA2 and TET2 to reestablish balanced GATA2 levels that permit leukemia development and progression. Fig. 7: TET2 lesions enhance the aggressiveness of CEBPA- mutant AML by rebalancing GATA2 expression. a Model of Gata2 differential expression as a consequence of (I) elevated CEBPA p30 due to the hypermorphic effect of the CEBPA NT , (II) TET2 deficiency and, (III) CEBPA deficiency. b Schematic illustration of two strategies for CEBPA DM AML to rebalance GATA2 levels by (I) loss-of-function mutations in TET2 and (II) loss-of-function mutations in one GATA2 allele. The illustrations were created with BioRender.com. Full size image Our work highlights the central importance of GATA2 regulation in CEBPA -mutant AML. Specifically, we show that GATA2 is a conserved target gene of CEBPA and TET2. Furthermore, the elevated levels of the CEBPA p30 variant likely mediate GATA2 upregulation in CEBPA-mutant AML. The increased expression of Gata2 is counteracted by loss of TET2 in vitro and in vivo models of Cebpa DM AML as well as in CEBPA - TET2 co-mutated patients. This is accompanied by the gain of Gata2 promoter DNA methylation. These findings are consistent with previous data showing that Gata2 expression is TET2-dependent, as Gata2 was downregulated in various Tet2 knockout settings and that forced expression of Gata2 decreased the competitiveness of both normal and malignant TET2-deficient cells [28] , [43] , [44] , [45] . Further paralleling our data, TET2 deficiency in the context of Flt3 ITD AML has been shown to accelerate leukemia by hypermethylation and consequent silencing of the Gata2 locus [43] . Strikingly, we found that while moderate reduction of Gata2 expression increased competitiveness in Cebpa DM AML both in vivo and in vitro, leukemia cells remain critically dependent on residual GATA2 function. Indeed, homozygous Gata2 lesions induced a strong inhibitory effect on Cebpa DM AML in vitro [37] , which was also observed in other AML subtypes as well as in normal hematopoietic stem cells [36] , [46] , [47] , [48] . These findings are corroborated by a substantial body of genetic evidence supporting the importance of GATA2 regulation in CEBPA -mutant AML. First, heterozygous GATA2 lesions frequently co-occur with CEBPA DM [4] , [8] , [16] , [17] , [31] , [32] , [33] , [49] , [50] , [51] , [52] . Secondly, GATA2 allele-specific expression is strongly associated with CEBPA DM AML and is neither found in AML with reduced CEBPA expression (i.e. t(8;21)) nor in CEBPA -silenced AML [53] . Thirdly, TET2 MUT and GATA2 MUT rarely co-occur in CEBPA DM AML. Finally, we showed that mutations in GATA2 and TET2 are overrepresented in AML cases with high CEBPA expression. This supports the notion that unfavorable, high GATA2 levels in AML promoted by the CEBPA-TET2 axis are not limited to CEBPA DM AML, but also include cases where CEBPA expression is high for other reasons. Further, this model also suggests that a major proleukemic effect of TET2 deficiency is to rebalance GATA2 levels in the context of CEBPA DM AML (see Fig. 7b ). GATA2 expression is mainly driven by the conserved G2 DHE in normal myeloid progenitors and leukemic blasts by promoting expression from the hematopoietic specific Gata2 V2 promoter [39] , [40] , [44] , [54] . Our data demonstrate that CEBPA plays a key role in regulating G2 DHE activity. Specifically, we showed that the hypermorphic effects of CEBPA DM [11] , and experimental models thereof, resulted in increased GATA2 expression compared to CEBPA WT , and that CEBPA deficiency resulted in reduced Gata2 levels. Secondly, we observed increased CEBPA binding to the G2 DHE in Cebpa DM AML compared to normal progenitors and found that deletion or mutagenesis of the CEBPA-bound region of the enhancer resulted in lower expression of Gata2 in Cebpa DM cells. In further support of the role of CEBPA, the G2 DHE is highly active in CEBPA DM AML, with both elevated eRNA expression and levels of H3K27ac [53] . An equally important role for CEBPA is observed in the context of inv(3) and t(3;3) AML in which inversions, translocations, and rearrangements involving the EVI1 gene at the MECOM locus , lead to hijacking of the G2 DHE to promote EVII expression at the expense of GATA2 expression thus resulting in GATA2 haploinsufficiency [55] , [56] , [57] , [58] . Here, EVI1 expression was found to be downregulated following knockdown of CEBPA in inv(3) AML cells, and mutation of the CEBPA binding site in the hijacked enhancer reduced enhancer activity [58] . In this context, CEBPA MUT would not be favorable, and these lesions are indeed underrepresented in inv(3) and t(3;3) AML [59] , [60] , [61] . We hypothesized that CEBPA recruits TET2 and thus mediates DNA demethylation of the Gata2 V2 promoter in a CEBPA- and TET2-dependent manner. Indeed, we observed reduced TET2-binding to the G2 DHE upon knockdown of Cebpa in Cebpa p30/p30 cells. Furthermore, Gata2 V2 levels were decreased, and Gata2 V2 promoter DNA methylation was increased upon Cebpa depletion in an MLL-AF9 leukemic setting where CEBPA is dispensable for maintenance of the leukemia. The concept of CEBPA as a recruiting factor for TET2 is also supported by previous findings showing that both the p30 and p42 isoforms of CEBPA interact with TET2 via the DNA binding domain of CEBPA [62] , [63] . Further, CEBPA binds preferentially to methylated DNA [62] , [64] , and has been classified as a binding site-directed DNA demethylation-inducing transcription factor [62] , [65] . Interestingly, TET2 binds genomic regions that are enriched for CEBP motifs in myeloid cells, particularly in myeloid enhancers such as the G2 DHE [26] , [62] . Moreover, knockdown or knockout of Tet2 leads to impaired upregulation of myeloid-specific genes upon Cebpa induction, with corresponding increased promoter methylation [66] . Also, in TET2 MUT or Tet2 −/− leukemia an enrichment of CEBP motifs at or near hypermethylated CpGs was observed [26] , [67] . Importantly, AML with silenced CEBPA is associated with DNA hypermethylation, a feature that is not present in CEBPA DM AML, which may suggest a broader function of CEBPA in the recruitment of TET2 [68] . In summary, we conclude that CEBPA plays an important role in the recruitment of TET2 to chromatin at the G2 DHE, promoting DNA demethylation at the Gata2 V2 promoter and the induction of Gata2 expression. The extent to which this can be extended to other loci warrants further analysis but is supported by the data mentioned above. While our findings suggest that GATA2 MUT and TET2 MUT both converge at rebalancing the increased expression of GATA2 in CEBPA DM AML, patients with CEBPA DM and GATA2 MUT have a more favorable prognosis [16] , [31] , [32] , [33] , [49] than patients harboring the CEBPA DM and TET2 MUT combination [16] , [17] . This suggests that while GATA2 deregulation plays an important role in leukemogenesis in the CEBPA MUT context, TET2 deficiency may likely contribute to malignancy through additional mechanisms that shall remain the subject of future work. Of clinical interest, we find that TET2 deficiency renders Cebpa DM AML sensitive to 5 - AZA and that TET2-deficient cells lose their proliferative advantage over TET2-proficient cells following 5-AZA treatment. In agreement with TET2-dependent Gata2 expression, ours and previous results show that 5-AZA treatment derepresses Gata2 expression in TET2-deficient cells [44] . Intriguingly, CEBPA CT mutations have recently been reported to sensitize AML to treatment with hypomethylating agents by disrupting the inhibitory interaction with DNMT3A mediated by the wild-type CEBPA bZIP domain [69] . Taken together, this suggests that demethylating agents could be a particularly interesting treatment option in CEBPA DM TET2 MUT patients. Finally, we note that although our mechanistic data have been acquired in experimental models of complete TET2 loss, data from AML patients indicates that TET2 haploinsufficiency is sufficient to rebalance GATA2 levels. We are also aware of the fact that our experimental models mimic AML in which the CEBPA p30 variant constitutes the sole CEBPA entity, which is different from the combination of N- and C-terminal mutations that constitutes the bulk of human CEBPA DM AML cases. However, since our main findings from the murine Cebpa p30/p30 / Cebpa Δ/p30 models are also observed in human CEBPA DM AML (including upregulation of CEBPA and GATA2 in leukemic GMPs compared to normal GMPs, as well as rebalancing of GATA2 expression and worsened outcome by the acquisition of TET2 lesions), we believe that our observations indicate that a similar disease-relevant CEBPA-TET2 axis is active in human CEBPA DM AML. In conclusion, our results reveal that GATA2 is a conserved target of the CEBPA-TET2 mutational axis in CEBPA DM AML and we propose an intricate mechanism by which elevated CEBPA p30 levels mediate recruitment of TET2 to regulatory regions of the Gata2 gene to promote its expression. We demonstrate that increased GATA2 levels are disadvantageous to CEBPA DM leukemic cells and that this can be counteracted by TET2 loss thus providing an explanation for the co-occurrence of CEBPA and TET2 lesions in AML. Finally, increased Gata2 promoter methylation, inflicted by TET2 deficiency, can be restored by demethylating 5-AZA treatment, thereby providing entry points for the development of rational targeted therapies in AML patients with these mutations. Patient data Assessment of mutational status To evaluate co-occurring mutations in CEBPA DM AML cases, data from published studies [3] , [4] , [5] , [6] , [7] , [8] , [17] including >40 CEBPA DM cases were extracted, and co-occurring mutations were evaluated (Supplemental Table 1 ). To determine frequencies of target gene mutations between CEBPA DM AML cases with TET2 MUT compared to TET2 wild-type ( TET2 WT ) AML cases, data from published studies [3] , [4] , [5] , [7] , [8] , [17] , [51] with specified mutational status including >40 CEBPA DM cases or corresponding cohorts were extracted and co-occurring mutations in TET2 , GATA2, WT1, CSF3R , and ASXL1 were evaluated (Supplemental Table 2a–e ). To examine how the mutational status of TET2 and GATA2 were affected by CEBPA expression levels in AML, we utilized the publicly available data from the Beat AML cohort (Oregon Health & Science University; OHSU) [1] , including 382 cases for which mutation and mRNA expression data were available. The cases were stratified based on CEBPA mRNA expression levels (z-score ±1.0 relative to all samples; CEBPA HIGH n = 45 and CEBPA LOW n = 61) and frequencies of CEBPA , TET2, and GATA2 mutations were determined. Survival analysis The clinical data set comprises 298 patients with CEBPA mutations (MLL Münchner Leukämielabor GmbH), of which 152 harbored biallelic CEBPA mutations. 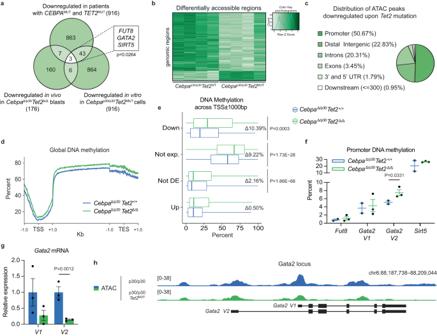Fig. 3: Loss of TET2 leads to reducedGata2levels inCebpa-mutant AML. aConserved targets of the CEBPA-TET2 axis visualized in a Venn-diagram of downregulated genes inCEBPA-TET2co-mutated AML overlaid with corresponding data fromTet2-deficient in vivo and in vitro models ofCebpaDMAML (P= 0.0264 vs. number of overlapping genes expected by random distribution assessed by Wilson/Brown binominal test).bHeatmap of differentially accessible regions assessed by assay for transposase-accessible chromatin sequencing (ATAC-seq; FDR < 0.05), andcgenomic distribution of downregulated peaks (FDR < 0.05, Log2FC < 0) uponTet2mutation (4 clones per group). Differential analysis was performed with DiffBind and region enrichment analysis with GREAT.dRepresentative genome wide DNA-methylation status in leukemic blasts from the in vivo model assessed by whole genome bisulfite sequencing (WGBS) showing frequency of methyl-cytosine (mC) across the transcription start site (TSS) ±1000 base pairs, gene body scaled to 4000 base pairs, and transcription termination site (TES) ±1000 base pairs. Methylation analysis was performed with Bismark and visualized using deepTools.eMedian and interquartile range of percent mC at promoters of down- (n= 172), not expressed (n= 6539), not differentially expressed (not DE; n = 14759) and up-regulated (n= 57) genes (averaged data generated from 2CebpaΔ/p30Tet2+/+and 3CebpaΔ/p30Tet2Δ/Δmice). Whiskers indicates max–min and data were analyzed by two-tailed unpairedt-test.fPromoter DNA methylation of conserved target genes in leukemic blast (samples from 2CebpaΔ/p30Tet2+/+and 3CebpaΔ/p30Tet2Δ/Δmice). Data are presented as mean±SEM. The data were log-transformed and analyzed by two-tailed unpairedt-test.gGata2variant mRNA expression inCebpaΔ/p30Tet2Δ/ΔandCebpaΔ/p30Tet2+/+leukemic blasts (samples from 3 mice per group). Data are presented as mean ± SEM. The data were log-transformed and analyzed by a two-tailed unpairedt-test.hSchematic genomic view of theGata2locus, including representative examples of assay for transposase-accessible chromatin using sequencing (ATAC-seq) inCebpap30/p30cells. Source data are provided as a Source Data file. Out of these 119 had specified TET2 mutational status and were included in the analyses ( CEBPA DM TET2 WT n = 84, CEBPA DM TET2 MUT n = 35; Supplemental Table 3 ). All patients gave written informed consent for the use of data for scientific evaluations. The study was approved by the Internal Review Board and by the Bavarian Ethics Committee, the Bavarian State Medical Association (Bayerische Landesärztekammer) with the number 05117. The study adhered to the tenets of the Declaration of Helsinki. Gene expression The Beat AML dataset used in this study is available at http://vizome.org/aml and comprises 25 patients with CEBPA mutations (CEBPA NT and/or CEBPA CT ) for which mutation and mRNA expression data is available. For the gene expression analysis, we excluded patients, which had co-occurring mutation(s) in WT1 or IDH1/2 since these have been shown to interfere with TET2 function [70] , [71] , [72] , [73] as well as two patients with low CEBPA variant allele frequency (VAF). 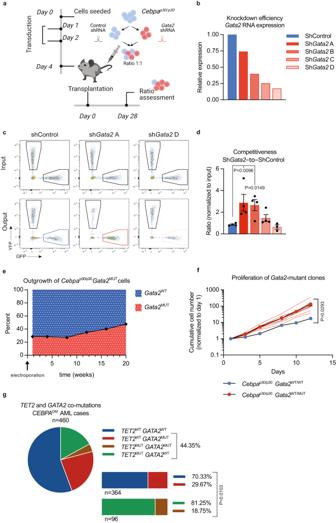Fig. 4: ModerateGata2reduction increases competitiveness ofCebpa-mutant AML. aExperimental setup for evaluating the effect ofGata2knockdown, via short hairpin RNA (shRNA) mediated silencing, onCebpap30/p30leukemic cells in a competitive in vivo assay. The illustration was created with BioRender.com.bGata2mRNA inCebpap30/p30leukemic cells prior to transplantation.cRepresentative flow cytometry profiles of input and output of shControl (no knockdown), shGata2A (low knockdown), and shGata2D (high knockdown).dCompetitive advantage of targeting shRNA (GFP+) vs. non-targeting shRNA (YFP+) cells in vivo assessed as by flow cytometry (Control 4, shGata2A 4, shGata2B 4, shGata2C 4, and shGata2D 3 mice). Data are presented as mean±SEM. Data were log-transformed and analyzed by one-way-ANOVA followed by Dunnett’s multiple comparisons correction.eExperimental setup forGata2CRISPR/Cas9 mutagenesis inCebpap30/p30cells, and outgrowth of heterozygous mutated clones. Percentages ofGata2mutated clones are indicated.fGrowth curve ofCebpap30/p30clones withGata2mutation (Cebpap30/p30Gata2+/MUT,n= 10) or wild typeGata2(Cebpap30/p30Gata2+/+,n= 3). Data are presented as mean±SEM and analyzed by two-tailed unpairedt-test. Red lines mark individual mutated clones.gPresence or absence ofGATA2mutations (GATA2MUT) inCEBPAdouble mutated (CEBPADM)AML cases with or withoutTET2mutations (TET2MUT) in aggregated data from published cohorts3,4,5,7,8,17(detailed in Supplemental Table2a). Data were analyzed by Wilson/Brown binominal test. Source data are provided as a Source Data file. Gene expression analysis was conducted on data from 16 CEBPA -mutant patients of which 5 have a co-occurring mutation in TET2 ( TET2 MUT ) (Supplemental Table 4 ). Differential expression analysis was performed with DESeq2 [74] (v. 1.26.0, RRID:SCR_015687) and default parameters. To assess gene expression changes in CEBPA WT patients with TET2 MUT vs TET2 WT , we included patients with normal karyotype AML from the Beat AML dataset and excluded patients with mutation(s) in WT1 or IDH1/2 (CEBPA WT TET2 MUT n = 34 and CEBPA WT TET2 WT n = 167). To analyze CEBPA and GATA2 expression levels in CEBPA WT vs. CEBPA NT AML mRNA expression of the two genes together with mutational and karyotype status data was retrieved from the Beat AML study [1] via cBioPortal [75] , [76] (RRID:SCR_014555). We evaluated patients for whom data was available for genomic profiling including mRNA expression, mutations, and karyotype. We included patients with normal karyotype AML and excluded patients with mutation(s) in WT1 or IDH1/2 ( CEBPA WT n = 52 and CEBPA NT n = 15). In vitro experiments Competitive CRISPR-targeting For generation of Tet2 or Gata2 mutated clones, Cebpa p30/p30 (♂) cells [37] were electroporated with ribonucleoparticles containing recombinant Cas9 nuclease from Streptococcus pyogenes (Sp) (#1081058, IDT), tracrRNA (#1075927, IDT) and crRNAs (Alt-R® CRISPR-Cas9 crRNA, IDT) targeting Tet2 and Gata2 , respectively. 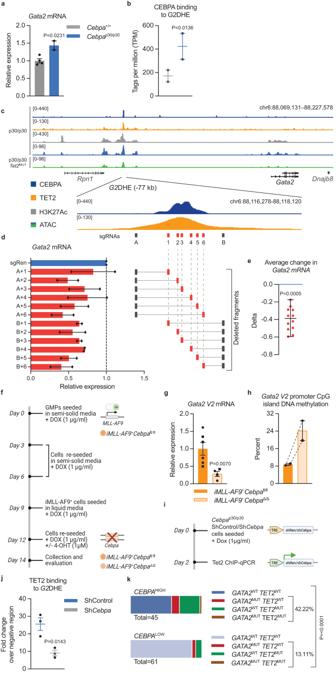Fig. 5: Increased CEBPA p30 binding to theGata2distal hematopoietic enhancer drives expression ofGata2via TET2. aGata2mRNA expression in mouseCebpap30/p30leukemic granulocyte/monocyte progenitors (GMPs) vs normal GMPs (samples from 4Cebpa+/+and 2Cebpap30/p30mice) and,bCEBPA binding to theGata2distal hematopoietic enhancer (G2DHE; −77 kb) region (samples from 2 mice per group), data from Jakobsen et al.11. Data are presented as mean ± SEM. Differential analysis was performed with DESeq2 (P< 0.05).cSchematic genomic view of theGata2distal hematopoietic enhancer (G2DHE), including normalized chromatin immunoprecipitation sequencing (ChIP-seq) signal of CEBPA (data from Heyes et al.12), TET2 and H3K27Ac (data from Heyes et al.12), as well as assay for transposase-accessible chromatin using sequencing (ATAC-seq) inCebpap30/p30cells without (light blue) and with (green) mutation inTet2.dGata2mRNA levels in response to targeting of theG2DHE by CRISPR-Cas9 inCebpap30/p30cells in vitro using indicated sgRNAs andethe averaged change inGata2mRNA levels of the 12 deletions (averaged data from 2 separate experiments). Data are presented as median ± range and analyzed by two-tailed Wilcoxon signed-rank test.fExperimental setup for evaluating the effects ofCebpaknockout onGata2 V2mRNA expression and DNA methylation of the CpG island at the promoter ofGata2 V2in MLL-fusion driven AML (iMLL-AF9). The illustration was created with BioRender.com.gGata2 V2mRNA expression (leukemic cell lines generated from 2 separate mice were assayed on 2 separate days in 2–3 technical replicates each). Data are presented as mean ± SEM and the individual cell lines are indicated by circles or squares. Data were log-transformed and analyzed by two-tailed unpairedt-test.hDNA methylation of theGata2V2 promoter CpG-island (2 separate leukemic cell lines). Data are presented as median±range and the individual cell lines are indicated by circles or squares.iExperimental setup for evaluating the effects ofCebpaknockdown on TET2 binding to theG2DHE inCebpap30/p30cells with inducible expression of shRNA targetingCebpaand control (Renilla), respectively. The illustration was created with BioRender.com.jTET2 binding to theG2DHE assessed by ChIP-qPCR (3 replicates per condition). Data are presented as mean±SEM and analyzed by two-tailed unpairedt-test.kFrequency ofGATA2and/orTET2mutations (GATA2MUTand TET2MUT, respectively) inCEBPAhigh expressing (CEBPAHIGH; 45 cases) vs.CEBPAlow expressing (CEBPALOW; 61 cases) AML cases, data from Beat AML cohort1. The distributions ofGATA2WTTET2WTvs.GATA2MUTand/orTET2MUTcases were analyzed by Wilson/Brown binominal test. Source data are provided as a Source Data file. crRNAs were designed using the CHOPCHOP [77] web tool (chopchop.cbu.uib.no, RRID:SCR_015723) (Supplemental Table 5 ). crRNA and tracrRNA molecules were complexed at room temperature and assembled with recombinant SpCas9 according to the manufacturer’s protocols (IDT). Pools of Tet2- or Gata2 -targeted cells were screened at regular intervals to monitor the outgrowth of subpopulations. The genomic regions that were targeted with CRISPR/Cas9 technology were PCR-amplified, Sanger sequenced, and analyzed with the online tool Tracking of Indels by DEcomposition (TIDE) [78] for insertions or deletions (indels) in the targeted region. 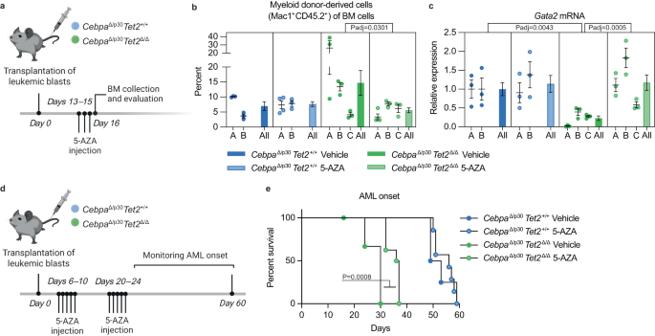Fig. 6: Demethylating treatment restoresGata2expression and prolongs survival in TET2-deficientCebpa-mutant AML. aExperimental setup for evaluating the effect of short-term 5-azacytidine (5-AZA) treatment in vivo. Recipient mice were sub-lethally irradiated and transplanted with leukemic BM from moribund secondary recipient mice. Three individualCebpaΔ/p30Tet2Δ/Δclones (A–C) and twoCebpaΔ/p30Tet2+/+clones (A–B) were used, respectively. The illustration was created with BioRender.com.bExpansion of myeloid (Mac1+) donor-derived cells in bone marrow (BM) assessed by flow cytometry, andcGata2mRNA expression in sorted leukemic blasts by qPCR assessed 24 hours after the last of three injections of 5-AZA or vehicle (samples from 3 mice per clone and 6 and 9 mice per group, forCebpaΔ/p30Tet2+/+ andCebpaΔ/p30Tet2Δ/Δ, respectively). Dot plots showing individual mice for separate clones and bar graphs shows mean ± SEM for each group. Data were analyzed by Kruskal–Wallis test followed by Dunn’s correction for multiple comparisons.dExperimental setup for evaluating the effect of 5-AZA treatment on AML progression in vivo. The illustration was created with BioRender.com.eSurvival of sub-lethally irradiated tertiary recipient mice after transplantation of leukemic BM from moribund secondary recipient mice (clone A from both genotypes) in response to intermittent 5-AZA treatment (5-AZA treated groups 8 mice and vehicle-treated groups 4 mice). The data were analyzed by Mantel–Cox Log-rank test. Source data are provided as a Source Data file. Primers for PCR are provided in Supplemental Table 6 . Gata2 enhancer CRISPR-targeting sgRNA sequences targeting the Gata2 distal hematopoietic enhancer (G2DHE) were obtained from the UCSC Genome Browser [79] (genome.ucsc.edu, RRID:SCR_005780) and targets with a high predicted cleavage (Doench/Fusi 2016 Efficiency > 55) [80] selected (Supplemental table 5 ). SpCas9-expressing Cebpa p30/p30 Tet2 MUT cells were isolated after lentiviral expression of lenti-Cas9-Blast (#52962 Addgene). Cebpa p30/p30 and Cebpa p30/p30 Tet2 MUT cells were co-transduced with pLenti-hU6-sgG2DHE_A/B-IT-PGK-iRFP and LentiGuide-sgG2DHE_1–6-Puro-IRES-GFP. GFP + iRFP670 + cells were sorted via fluorescence-activated cell sorting (FACS) and frozen for subsequent analysis. Cebpa shRNA-knockdown Cepba p30/p30 rtTA3 cells expressing Dox-inducible shRNAs against Renilla luciferase (shRen, control) or Cebpa (sh Cebpa ) were used as previously described [12] . Cebpa knockdown was induced by the addition of 4-hydroxytamoxifen (4-OHT; 1 μM; #H7904 Sigma-Aldrich) to the cell culture medium to activate shRNA expression (mean Cebpa knockdown efficiency > 90% compared to shRen control) and cells were collected for further analysis after 48 h. In vivo experiments Experiments were carried out according to protocols approved by the Danish Animal Ethical Committee. Mice were bred and housed locally at the Department of Experimental Medicine at the University of Copenhagen. The mice were housed in a temperature- and humidity-controlled room with a 06:00–18:00 h light cycle and fed a standard chow diet and tap water ad libitum . We used Tet2 fl/fl [81] , Cebpa p30/+ [13] , Cebpa +/fl [82] and Mx1-Cre + [83] lines to generate inducible Tet2 -deficient and Cebpa -mutant compound lines. The following genotypes were used for experiments: Cebpa fl/p30 Tet2 +/+ , Cebpa +/fl Tet2 fl/fl , Cebpa fl/p30 Tet2 fl/fl , Cebpa fl/p30 Tet2 +/+ Mx1-Cre + , Cebpa +/fl Tet2 fl/fl Mx1-Cre + , and Cebpa fl/p30 Tet2 fl/fl Mx1-Cre + . Cebpa p30/p30 embryos were generated as previously described [13] . We used iMLL-AF9 + [84] , Cebpa +/fl [82] and R26-CreER + [85] lines to generate an iMLL-AF9 + Cebpa fl/fl R26-CreER + compound line. Primers for genotyping in are provided in Supplemental Table 6 . During the leukemia initiation and propagation experiments described below, the animals were monitored daily and euthanized when they showed sign(s) of sickness e.g., inactivity, hunched posture, white paws, and/or matted or puffed-up fur as well as pain assessed based on the NC3R’s mouse grimace scale [86] or reduced bodyweight (maximal allowed reduction = 15%). The experiments were terminated after 12 months. Leukemia initiation (Cebpa Δ/p30 model) C57BL/6 J.SJL congenic recipients (female, 10–12 weeks old) were lethally irradiated (900 cGy) 12–24 h prior to intravenous injection with 1 × 10 6 bone marrow (BM) cells from individual donor mice. The mice were given Ciprofloxacin (100 mg/l in acidified water; #17850 Sigma-Aldrich) in the drinking water to prevent infections 3 weeks post-irradiation. Recipient mice were allowed to recover for 6 weeks post-transplantation before Cre-LoxP recombination was induced by two intraperitoneal injections of Poly(I)-Poly(C) (300 μg in 200 μl PBS; #27-4732-01 GE Healthcare) with 48 h rest in-between. The day of the first injection was set as time-point zero for the survival study and mice were monitored for leukemia development and euthanized when moribund. To follow leukemia initiation in the recipients, a subgroup of mice was subjected to blood and BM sampling at 12, 24, and 36-week time-points. BM from moribund mice was collected and frozen (10% DMSO in FBS; #D8418 Sigma-Aldrich, #HYCLSV30160.03 Hyclone) for subsequent FACS and analysis. Leukemia initiation (Cebpa p30/p30 model) C57BL/6 J.SJL congenic recipients (female, 10 weeks old) were lethally irradiated (900 cGy) 12–24 h prior to intravenous injection with 0.5-1 × 10 6 fetal liver cells from E15.5 Cebpa p30/p30 embryos. The mice were given Ciprofloxacin (100 mg/l in acidified water) in the drinking water to prevent infections 3 weeks post-irradiation. Latency to leukemic initiation was 8-11 months. Leukemia propagation C57BL6/6 J.SJL recipients (female, 10–12 weeks old) were lethally irradiated (900 cGy) 12–24 h prior to being intravenously injected with 2 × 10 5 thawed live BM cells from moribund donor mice together with 4 × 10 5 freshly isolated BM cells from C57BL6/6 J.SJL mice. The day of the injection was set as time-point zero for the survival study and mice were monitored and euthanized when moribund. The mice were given Ciprofloxacin in the drinking water to prevent infections 3 weeks post-irradiation. Competitive shRNA-knockdown C57BL/6 J.SJL recipients (female, 10–12 weeks old) were sub-lethally irradiated (500 cGy) 12–24 h prior to being intravenously injected with a 1:1 mix of Cebpa p30/p30 cells [13] transduced with shRNA targeting Gata2 (detailed in ShRNA knockdown below) or with control-shRNA [87] . The ratio of Gata2 - or control-shRNA-GFP + to control-shRNA-YFP + cells was analyzed by flow cytometry four weeks later. 5-azacytidine treatment C57BL/6 J.SJL recipients (female, 10–12 weeks old) were sub-lethally irradiated (500 cGy) 12–24 h prior to being intravenously injected with 1 × 10 5 thawed live BM cells from moribund secondary recipient mice. The mice were given Ciprofloxacin in the drinking water to prevent infections 3 weeks post-irradiation. The mice received intraperitoneal injections with the demethylating agent 5-azacytidine (2.5 mg/kg/day in saline; #A2385 Sigma-Aldrich) at days 6–10 and 20–24 post-transplantation. The time of the BM cell injection was set as time-point zero for the survival study and mice were monitored and euthanized when moribund. To evaluate the effects of short-term 5-azacytidine treatment, recipient mice were treated at days 13–15 and euthanized 24 h after the last injection. BM was collected for FACS, and sorted cells were frozen for subsequent analysis. Ex vivo cell culture Establishment of ex vivo Cebpa Δ/p30 Tet2 +/+ and Cebpa Δ/p30 Tet2 Δ/Δ lines Thawed cryo-preserved cells from primary AML were cultured in Lonza X-Vivo TM 15 cell medium (#BE02-060Q Thermo Fisher Scientific) supplemented with Bovine Serum Albumin in Iscove’s MDM (10%; #09300 Stemcell TM Technologies), Penicillin-Streptomycin (1%; #15140122 Gibco), β-mercaptoethanol (0.1 mM; #31350010 Gibco), L-glutamine (2 mM; #25030149 Gibco), and cytokines h-IL-6 (50 ng/ml; #130-093-032 Miltenyi Biotec), m-SCF (50 ng/µl; #250-03 Peprotech), m-IL-3 (10 ng/ml; #213-13 Peprotech), and m-GM-CSF (10 ng/ml; #315-03 Peprotech). Two clones of each genotype ( Cebpa Δ/p30 Tet2 +/+ and Cebpa Δ/p30 Tet2 Δ/Δ ) continued to expand beyond 40 days and withstood freeze-thawing, and these clones have been used for further experiments. Vitamin C treatment Cells were seeded at a density of 2 × 10 5 cells/ml and the cell culture medium was supplemented with vitamin C (100 μg/ml; L-ascorbic acid, #A8960 Sigma Aldrich). Live cells were counted using Solution 13 (AO-DAPI; #910-3013 Chemometec) on a NucleoCounter® NC-3000 TM and reseeded at 2 × 10 5 cells/ml every third day. The experiments were run with a total of two biological replicates per genotype (performed on separate days) where each experiment assayed one leukemic line per genotype. Each condition (Vitamin C and vehicle) was performed in technical triplicates for each of the two biological replicates per genotype. 5-azacytidine treatment Cells were seeded at a density of 2 × 10 5 cells/ml and medium supplemented with 5-azacytidine (5-AZA; 1 μg/ml; #A2385 Sigma-Aldrich). Live cells were counted using Solution 13 on a NucleoCounter® NC-3000 TM and reseeded at 2 × 10 5 cells/ml days three and six. 24 hours later, up to 1 × 10 5 cells were isolated and resuspended in RA1 buffer (NucleoSpin RNA XS, #740902 Macherey-Nagel). The experiments were run with a total of two biological replicates per genotype (performed on separate days) where each experiment assayed one leukemic line per genotype. Each condition (5-AZA and vehicle) was performed in technical triplicates for each of the two biological replicates per genotype. Establishment of ex vivo iMLL-AF9 + Cebpa fl/fl R26-CreER + lines Sorted GMPs from iMLL-AF9 + Cebpa fl/fl R26CreER + mice, were cultured in MethoCult (M3434; #03434, Stemcell technologies) supplemented with doxycycline (1 μg/ml; #D9891 Sigma-Aldrich) for three replatings to induce expression of the MLL-fusion protein. Cebpa knockout Leukemic iMLL-AF9 + Cebpa fl/fl R26CreER + cells were cultured in RPMI 1640 medium (#21875034, Gibco) supplemented with FBS (10%), Penicillin-Streptomycin (1%), doxycycline (1 μg/ml), and cytokines m-IL-3 (6 ng/ml), m-SCF (50 ng/ml), and h-IL-6 (10 ng/ml). After two days, 4-hydroxytamoxifen (4-OHT; 1 μM; #H7904 Sigma-Aldrich) or vehicle was added to the cell culture medium to activate Cre-LoxP recombination, resulting in a reduction of Cebpa mRNA to 1.7 ± 0.3% vs. 100 ± 12.3% in vehicle control. Three days later cells were isolated and either frozen or resuspended in RA1 buffer (NucleoSpin RNA XS, # 740902 Macherey-Nagel). The experiments were run with a total of two biological replicates (performed on separate days). Each condition (4-OHT and vehicle) was performed in 2-3 technical triplicates for each of the two biological replicates. ShRNA knockdown Cloning of shRNA into pMLS vector Murine shRNAs targeting Gata2 (sh Gata2 ) were cloned into MSCV-LTRmir30-SV40-GFP vector. 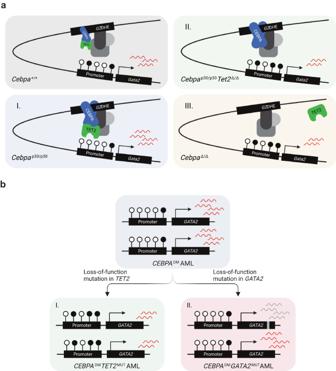Fig. 7:TET2lesions enhance the aggressiveness ofCEBPA-mutant AML by rebalancingGATA2expression. aModel ofGata2differential expression as a consequence of (I) elevated CEBPA p30 due to the hypermorphic effect of theCEBPANT, (II) TET2 deficiency and, (III) CEBPA deficiency.bSchematic illustration of two strategies forCEBPADMAML to rebalanceGATA2levels by (I) loss-of-function mutations inTET2and (II) loss-of-function mutations in oneGATA2allele. The illustrations were created with BioRender.com. Targeting sequences were identified from the Mission® shRNA library (Supplemental Table 7 ) and the sense and anti-sense sequences were incorporated with a miR-30-loop to generate a 97-mer target sequence. Oligonucleotides were amplified by PCR using miR30 common primers (Supplemental Table 6 ), which include restriction sites for XhoI and EcoRI . The resulting 138-mer PCR amplicons and the vector were digested with XhoI and EcoRI and products were ligated using T4 DNA Ligase (#15224025 Invitrogen). Bacterial transformation was performed to amplify individual ligation products, and correct inserts were verified by Sanger Sequencing. These, together with vectors containing a control non-targeting sequence (MSCV-LTRmir30-SV40-GFP and MSCV-LTRmir30-SV40-YFP), were used in subsequent transfection/transduction experiments, as previously described [87] , [88] . Transduction of Cebpa p30/p30 cells Retroviral transduction was done as previously described [87] . Briefly, retroviral supernatants were generated by transfection of Phoenix-Eco cells (RRID:CVCL_H717). For transduction, retroviral supernatant was added onto retronectin-coated (1:25; #T100B TaKaRa) non-tissue culture treated plates and centrifuged at 2000 ×g for 60 min at 4 °C. After aspiration of the supernatant, Cebpa p30/p30 cells were seeded at a density of 0.5–1 × 10 5 cells/cm 2 . The transduction was repeated the following day, and the cells were cultured for 24 h prior to FACS sorting of transduced (GFP + /YFP + ) cells on a BD FACSAria TM III (BD Bioscience). The efficiency of shRNA-mediated gene expression knockdown was assessed with qPCR and cells were used for transplantation and assessment of their competitiveness in vivo. Immuno-staining Flow cytometry To analyze the composition of either freshly isolated or thawed cryopreserved BM and blood, cells were stained with fluorescently labelled antibodies. For blood analysis, 50 µl blood was collected from the facial vein and erythrocytes were lysed with lysing buffer (BD Pharm Lyse TM , #555899 BD Bioscience). For BM analysis, cells were collected by crushing tibia, femur, and ilium and filtered through a 50 μm filcon cup (#340630 BD Bioscience). Blood or BM cells were washed in PBS with 3% FBS and stained with fluorescently labelled antibodies for 30 min at 4 °C (Supplemental Table 8 ). For cryopreserved cells, the cells were counterstained with DAPI (1:10000; #D3571 Invitrogen) to separate out dead cells. Fluorochrome-minus-one was used as controls. Flow cytometry data was obtained using a BD FACSAria TM III or a BD LSR II TM (BD Bioscience) and analyzed using FlowJo software (v9, RRID:SCR_008520). For downstream transcriptional and epigenetic analyses, live donor-derived non-lymphoid and non-erythroid cells (DAPI − CD45.2 + CD3 − B220 − Ter119 − ) were sorted using a BD FACSAria TM III, spun down and cell pellets were either snap-frozen or resuspended in RLT buffer (RNeasy Mini Kit, #74104 Qiagen). For ex vivo cell culture of iMLL-AF9 + Cebpa fl/fl R26-CreER + cells, c-kit + BM cells were enriched by magnetic sorting (mouse CD117 MicroBeads; #130-091-224, Miltenyi Biotec), and granulocyte/monocyte progenitors (GMPs; Lin − C-kit + Sca1 − CD41 − FcgRII + ) were sorted using a BD FACSAria TM III. Immunohistochemistry To evaluate the proliferative status of leukemia cells, cells from BM of moribund mice were spun on glass slides, air-dried, and fixed with methanol (#VWRC20846.292 VWR). After blocking of endogenous peroxidase activity with hydrogen peroxide (1%), slides were stained overnight at 4 °C with anti-Ki67 antibody (1:50; Clone SP6, RRID:AB_302459, #ab16667 Abcam) in antibody diluent (S3022 Dako). To visualize the primary antibody, EnVision HRP Rabbit (K4003 Dako) together with Vina Green TM Chromogen Kit (BRR807 Biocare Medical) was utilized according to manufacturer’s instructions. The cells were counterstained with Mayer Hematoxylin (#51275 Sigma-Aldrich), dehydrated and coverslips mounted with Entellan (#107960 Sigma-Aldrich). Images were captured using a Leica microscope at 20X magnification and Ki67 + cells were quantified out of one hundred cells. Western blotting Western blotting for TET2 was performed according to standard laboratory protocols, using the following antibodies: anti-TET2 (1:100, Clone C-7, RRID:AB_2924805, #sc-398535 Santa Cruz) and anti-HSC70 (1:10000, Clone B-6, RRID:AB_627761, #sc-7298 Santa Cruz). Quantitative PCR RNA from sorted blasts or ex vivo-cultured cells was isolated using NucleoSpin RNA XS kit (#740902 Macherey-Nagel) or RNeasy Mini Kit (#74104 Qiagen) according to the manufacturers’ instructions and converted to cDNA using ProtoScript First Strand cDNA Synthesis Kit (#E6300 New England BioLabs). Quantitative PCR (qPCR) to assess knockdown efficiency was run using TaqMan Fast Advanced Master Mix (#4444556 Applied Biosystems) and TaqMan assay for Gata2 (Mm00492301_m1 FAM-MGB), in duplex with housekeeping gene 18 S (Hs99999901_s1 VIC-MGB-PL). TaqMan assay for Ki67 (Mm01278617_m1 FAM-MGB) was used to assess the expression of the proliferation marker. qPCR to evaluate mRNA levels of total Gata2 , variant 1 ( V1 ) and variant 2 ( V2 ), respectively, was run in duplex using LightCycler 480 SYBR Green I Master (#04887352001 Roche) with primers for Gata2 and housekeeping gene Actb and Gapdh [41] (Supplemental Table 6 ). Gene expression was calculated with the 2 −ΔΔct method. RNA from Cebpa p30/p30 cell lines was isolated using RNeasy Plus Mini Kit (#74134 Qiagen) according to the manufacturer’s instructions and converted to cDNA with RevertAid First Strand cDNA Synthesis Kit (#K1622 Thermo Scientific). qPCR was run using SsoAdvanced Univ SYBR Grn Suprmix (#1725271, Bio-Rad Laboratories Ges.m.b.H.) and primers for Gata2 and Gapdh (Supplemental Table 6 ). Bisulfite PCR DNA was isolated using DNeasy Blood and tissue kit (#69504 Qiagen) and the DNA was bisulfite converted using EZ-DNA Methylation Gold Kit (#D5005 Zymo Research), both according to the manufacturer’s instructions. PCR was run using Pfu Turbo Cx Hotstart DNA polymerase (#600410 Agilent) with primers targeting a part of the CpG island in the Gata2 V2 promoter region (Supplemental table 6 ). After verification of their correct size, PCR products were cloned using Zero Blunt Topo PCR Cloning kit (#450245 Invitrogen), and single colonies were picked and amplified. Plasmid DNA was isolated using NucleoSpin Plasmid EasyPure (#740727.250 Macherey-Nagel), the correct insert size was verified after cleavage with restriction enzyme EcoRI (#R0101 New England Biolabs) and sent for Sanger sequencing using the M13 primer provided with the cloning kit. Chromatin immunoprecipitation (ChIP)-qPCR ChIP for CEBPA was performed as previously described [37] using an anti-CEBPA antibody (1:60, C-18, RRID:AB_2078046, #sc-9314, Santa Cruz Biotechnology). ChIP for TET2 was performed using an anti-TET2 antibody (1:50; clone D6C7K, RRID:AB_2799102, #36449, Cell Signaling Technology), as previously described [37] , including a 30-minute incubation with 2 mM disuccunumidyl glutarate (DSG; #20593 Thermo Scientific) before the 1% formaldehyde crosslinking step. The sequences used for qPCR are listed in Supplemental table 6 . High-throughput sequencing and bioinformatic analyses RNA-sequencing (RNA-seq) of cell line models RNA was isolated from 1 × 10 6 cells using RNeasy Plus Mini Kit (#74134 Qiagen) according to the manufacturer’s instructions and quality was assessed on a Bioanalyzer 2100 G2939A (Agilent). 1 µg of RNA was used to generate sequencing libraries using QuantSeq 3′ mRNA-Seq Library Prep Kit (FWD) for Illumina, 96 preps (#015.96, Lexogen) and the PCR Add-on Kit for Illumina, 96 rxn (#020.96, Lexogen). The libraries were quantified on a Bioanalyzer 2100 G2939 (Agilent) and pooled in equimolar amounts. Multiplexed libraries were sequenced on a HiSeq4A (Illumina). RNA-seq of leukemic cells from in vivo models RNA was isolated from 5 × 10 5 sorted cells using RNeasy Mini Kit (#74104 Qiagen) according to the manufacturer’s instructions and quality was assessed by RNA 6000 Pico Kit (#5067-1513 Agilent) on a Bioanalyzer 2100 (Agilent). 200 ng RNA was used to generate sequencing libraries using TruSeq RNA Library Prep Kit v2 (#RS-122-2001 Illumina). The libraries were quantified using Qubit dsDNA BR Assay Kit (#32853 Thermo Fisher Scientific) and DNA 1000 Kit (#5067-1504 Agilent) and pooled in equimolar amounts. Multiplexed libraries were sequenced on a NextSeq 500 (Illumina) using NextSeq 500 High Output v2 Kit (75 cycles; #FC-404-2005 Illumina). Bioinformatics analyses of RNA-seq data RNA-seq analysis for in vitro Cebpa p30/p30 cells was performed as previously described [12] , [37] . Quality check was done with FastQC [89] (v. 0.11.4, RRID:SCR_014583) and preprocessing with PRINSEQ-lite [90] (v. 0.20.4; RRID:SCR_005454), using parameters: -min_len 30 -min_qual_mean 30 -ns_max_n 5 -trim_tail_right 8 -trim_tail_left 8 -trim_qual_right 30 -trim_qual_left 30 -trim_qual_window 5. The remaining reads were aligned against the mouse reference genome (mm10) with BWA [91] (v. 0.7.15; RRID:SCR_010910). RNA-seq analysis for in vivo Cebpa Δ/p30 cells was performed as follows. RNA-seq reads were processed with the bcbio RNA-seq pipeline [92] ( https://github.com/bcbio/bcbio-nextgen , RRID:SCR_004316) and the bcbioRNASeq R package ( https://github.com/hbc/bcbioRNASeq ). In brief, transcript abundance estimates were obtained using Salmon [93] (v. 0.12.0, RRID:SCR_017036) against reference transcriptome GRCm38/mm10 ENSEMBL release 94, summarized to gene level and imported into R using tximport [94] (v. 1.10.1, RRID:SCR_016752) (using setting countsFromAbundance = “lengthScaledTPM”). Differential gene expression analysis between the Cebpa Δ/p30 Tet2 +/+ and Cebpa Δ/p30 Tet2 Δ/Δ genotype was performed using DESeq2 with standard parameters [74] (v. 1.22.2, RRID:SCR_015687) excluding lowly expressed genes ( < 10 sum normalized counts across all samples) and running with alpha = 0.05. Gene expression levels between primary Cebpa Δ/p30 Tet2 +/+ and established Cebpa p30/p30 leukemias were compared using edgeR (v. 3.32.1, RRID:SCR_012802). Gene set enrichment analysis (GSEA) GSEA was performed using the GSEA software [95] , [96] (v. 4.1.0, RRID:SCR_003199) and the Molecular Signatures Database (RRID:SCR_016863). Assay for transposase-accessible chromatin-sequencing (ATAC-seq) ATAC-seq was performed as previously described [12] . Bioinformatics analyses of ATAC-seq data Analysis of ATAC-seq was performed as previously described [12] . HOMER [97] (v. 4.11, RRID:SCR_010881) was used to identify motifs enriched in the ATAC peaks. Bisulfite whole genome sequencing (WGBS) DNA was isolated from 1 × 10 6 sorted cells using DNeasy Blood and tissue kit (#69504 Qiagen) according to the manufacturer’s instructions. Bisulfite conversion of DNA was done according to manufacturers’ instructions using EZ-DNA Methylation Gold Kit (#D5005 Zymo Research). Quality of bisulfite treated DNA was assessed by RNA 6000 Pico Kit (#5067-1513 Agilent) on a Bioanalyzer 2100. Libraries of bisulfite-converted DNA were prepared using Pico Methyl-Seq Library Prep Kit (#D5455 Zymo Research) according to manufacturer’s instructions and the final concentration and quality of the libraries was assessed using Qubit dsDNA HS Assay Kit (#Q32854 Thermo Fisher Scientific) and High Sensitivity DNA Analysis Kit (#5067-4626 Agilent) on a Bioanalyzer. Duplexed libraries were sequenced on a NextSeq 500 (Illumina) using NextSeq 500 High Output v2 Kit (75 cycles). Bioinformatics analyses of WGBS data Reads were trimmed and filtered using Trim Galore [98] (v. 0.4.3, RRID:SCR_011847) with default parameters, and quality was assessed before and after using FastQC [89] (v. 0.11.7). Trimmed reads were aligned to the mouse genome assembly GRCm38 (mm10) using Bismark [99] (v. 0.19.1, RRID:SCR_005604) with option -non_directional (other parameter left at default values; this used Bowtie 2 [100] (v. 2.2.8 RRID:SCR_016368) with -q --score-min L,0,−0.2 --ignore-quals). After deduplication of alignments (using deduplicate_bismark), the methylation information for individual cytosines was extracted using bismark_methylation_extractor (--cytosine_report --comprehensive --gzip). To quantify DNA methylation of gene bodies and promoters (1000 bp up-and downstream of transcription start sites), we used the weighted methylation level (i.e., summarizing over all CpG positions in the given region, the number of reads supporting methylated cytosine divided by the number of all reads covering these positions). Plots of average methylation levels across extended gene bodies were generated using deepTools [101] (v.3.1.3, RRID:SCR_016366) computeMatrix (scale-regions -m 4000 -a 1000 -b 1000 --unscaled5prime 1000 --unscaled3prime 1000) and plotProfile, for which Bismark-generated bedGraph files were converted to BigWig format (using UCSC’s bedGraphToBigWig [102] (v. 4)). Bioinformatic analyses of chromatin immunoprecipitation-sequencing (ChIP-seq) ChIP-seq data from in vitro Cebpa p30/p30 cells was processed as described [12] . ChIP-seq data from in vivo Cebpa p30/p30 cells was processed as follows; raw reads derived from CEBPA ( Cebpa +/+ and Cebpa p30/p30 ) ChIP-seq experiments were mapped to mouse (mm10) genome assembly using Bowtie 2 [100] (v. 2.3.4.3). We used uniquely mapped and PCR duplicates (exact copies) collapsed as one read and extended to their fragment length by determining the read extension size using MACS2 [103] (v. 2.1.0.20151222; predicted parameter, RRID:SCR_013291). Raw read counts were normalized to TPM using deepTools [101] (v. 3.3.1; bamCoverage). Raw read counts (CEBPA binding levels) mapping to Gata2 promoter and enhancer regions were computed using bedtools [104] (v. 2.30.0; multicov, RRID:SCR_006646), and the differences in CEBPA binding between Cebpa +/+ and Cebpa p30/p30 conditions were computed using DESeq2 [74] (v. 1.30.1). Sequencing reads derived from TET2 ChIP-seq experiment were preprocessed with PRINSEQ-lite [90] (v. 0.20.4; RRID:SCR_005454) and the remaining reads were mapped to the mouse reference genome sequence (mm10) using BWA [91] (v. 0.7.17-r1188, RRID:SCR_010910). The resulting alignments were processed with samtools [105] (v. 1.13; RRID:SCR_002105) and peak calling was done with MACS2 [103] (v. 2.1.0.20140616; RRID:SCR_013291). Aligned read counts were normalized to RPKM using the bamCoverage function from deeptools [101] (v. 3.5.1; RRID:SCR_016366). Statistics Data were analyzed for significance using parametric tests, with prior log-transformation if necessary to achieve normal distribution. Normality was evaluated by Shapiro–Wilk test. Two-group analyses were done using an unpaired two-tailed t -test. Multiple-group analyses were done with one-way-ANOVA followed by multiple comparisons correction using Dunnett when comparing to a reference group, or two-way-ANOVA followed by multiple comparisons correction using Šídák test when comparing two independent factors across four groups. Data sets that did not pass normality tests were analyzed by Kruskal–Wallis test followed by multiple comparisons correction using Dunn’s test. Survival curves were analyzed using Mantel–Cox Log-rank test. To compare distributions Wilson/Brown binominal test was used. To compare a median against a hypothetical median Wilcoxon signed-rank test was used. p -values < 0.05 were considered statistically significant. Data was analyzed using GraphPad Prism (v. 9, RRID:SCR_002798). Data is shown as mean ± SEM unless otherwise stated. Reporting summary Further information on research design is available in the Nature Portfolio Reporting Summary linked to this article.